Solid frustrated-Lewis-pair catalysts constructed by regulations on surface defects of porous nanorods of CeO2 Identification on catalytic sites of heterogeneous catalysts at atomic level is important to understand catalytic mechanism. Surface engineering on defects of metal oxides can construct new active sites and regulate catalytic activity and selectivity. Here we outline the strategy by controlling surface defects of nanoceria to create the solid frustrated Lewis pair (FLP) metal oxide for efficient hydrogenation of alkenes and alkynes. Porous nanorods of ceria ( PN -CeO 2 ) with a high concentration of surface defects construct new Lewis acidic sites by two adjacent surface Ce 3+ . The neighbouring surface lattice oxygen as Lewis base and constructed Lewis acid create solid FLP site due to the rigid lattice of ceria, which can easily dissociate H–H bond with low activation energy of 0.17 eV. Catalytic hydrogenation of unsaturated substrates, a fundamental transformation process, is finding prolific industrial reactions, especially for petrochemistry [1] , [2] , [3] . Hydrogen activation by either transition metal complexes or metal-based heterogeneous catalysts have been well developed and successfully applied for various reactions [4] . Recently, frustrated Lewis pairs (FLPs), Lewis acids and bases that are sterically prevented from interaction to form Lewis acid–base adjuncts, can efficiently and cooperatively activate many small molecules (for example, H 2 , CO 2 , and NO) and even strong C–H bond for important catalytic reactions including hydrogenation, hydroamination and carbon dioxide reduction [5] , [6] , [7] , [8] , [9] , [10] , [11] , [12] , [13] , [14] , [15] , [16] , [17] , [18] , [19] , [20] , [21] , [22] , [23] , [24] , [25] . However, molecular-based homogeneous FLP catalytic systems raise the difficulties in product purification and catalyst recovery. Therefore, the development of heterogeneous catalysts with FLP-like activity is extremely expected. Meanwhile, the combination of Au powder as Lewis acid and molecular Lewis bases (for example, imine and nitrile) successfully constructs the first example of semi-heterogeneous FLP catalytic system [26] . In this catalytic system, large quantity of Lewis acids and bases were required to avoid the formation of stable Lewis acid–base complexes. The semi-heterogeneous molecular sieves/B(C 6 F 5 ) 3 FLPs deliver remarkable catalytic activity for hydrogenation of ketones and aldehydes [27] . Graphene synthesized by chemical exfoliation has been reported as efficient catalysts for hydrogen activation through an FLP-like behaviour [28] . When the Lewis acid and base sites are in an adequate distance, the activation of hydrogen becomes possible [29] , [30] , [31] . However, they require restricted demanding reaction conditions with long reaction time and a high H 2 pressure of 30 bar [28] . Formation of an FLP of the Na + H − /hydroxyl proton O(H + ) has been successfully demonstrated for Pt x /NaY zeolites by using in situ neutron diffraction and spectroscopic measurements [32] . Inspired by the catalytic mechanism of molecular FLP catalysts, it is also possible to develop novel heterogeneous FLP-like catalysts if independent Lewis acidic and basic species coexist in one material. Recently, Ozin and colleagues [33] , [34] , [35] , [36] , [37] has reported that the surface FLP sites of In 2 O 3- x (OH) y created by a Lewis acidic coordinately unsaturated surface indium site proximal to an oxygen vacancy and a Lewis basic surface hydroxide site showed the catalytic activity for the CO 2 reduction by H 2 in both experimental results and theoretical predictions. It provides a possible strategy to construct solid FLP sites in oxides by creating oxygen vacancy. Nanostructured ceria is characterized with a large number of surface-bound defects that are primarily oxygen vacancy or Ce 3+ species as active sites for heterogeneous catalysis [38] , [39] , [40] , [41] , [42] , [43] . In previous investigations, the catalytic ability of ceria is driven by the ability to switch between different oxidation states (Ce 3+ /Ce 4+ redox pair) accompanied with the storage and release of oxygen when the temperature is higher than 150 °C (ref. 44 ). At low temperature, the surface oxygen is less mobile and can be firmly held in the lattice matrix [45] , [46] . With these precedents in mind, the combination of the ‘fixed’ surface oxygen as Lewis base and surface defects as Lewis acid in ceria is similar to the sterically encumbered pairs of Lewis acids and bases for molecular FLP catalysts, if the surface Lewis acid and base are independent. We choose ceria as another candidate to demonstrate the possibility to construct FLP sites due to its reversible Ce 3+ /Ce 4+ redox pair and rich surface chemistry [38] . Ceria has been reported to exhibit the catalytic activity for the selective semi-hydrogenation of alkynes through the H 2 activation by homolytic or heterolytic pathway and subsequent hydrogenation [47] , [48] , [49] , [50] , [51] . In general, a high temperature is required due to the inherent difficulty of ceria for H 2 activation. Heterolytic (between lattice Ce 4+ and O 2− ) pathway is considered as the pathway for H 2 dissociation due to the relative low activation energy [51] . Hence, it is not surprise to observe the decreased hydrogenation activity of ceria with the increased surface defects [47] , [49] . Incapability for hydrogenation of alkenes and restricted reaction conditions for semi-hydrogenation of alkynes indicate the low hydrogenation activity of ceria. In this work, solid FLP sites on CeO 2 surface, which deliver a very high catalytic activity for hydrogenation of alkenes and alkynes with a wide scope under mild conditions ( T =100 °C and P (H 2 )=1.0 MPa), have been successfully created by regulating their surface defects. The richness of surface defects is found to be the key for construction of a new surface Lewis acidic center by two adjacent reduced surface Ce atoms near an oxygen vacancy. The ‘fixed’ surface lattice oxygen as Lewis base and constructed Lewis acid have a large possibility to be close enough but independent due to the richness of surface defects and unique geometrical and electronic configurations, similar to the molecular-based FLPs. Porous nanorods of ceria ( PN -CeO 2 ) with a large surface Ce 3+ fraction of 30.8% associated with a high concentration of oxygen vacancy have been demonstrated as the solid metal oxide FLP catalyst with a low activation barrier of 0.17 eV for H 2 dissociation. Design strategy of solid FLP catalysts Metal oxides possess the surface Lewis acid (metal cation) and Lewis base (oxygen anion), which form the Lewis acid-base adjuncts and deliver no FLP-like activity [51] , [52] . Fortunately, the surface defects induced by the reducible/oxidable valence states of metal cations associated with oxygen vacancy in metal oxides can create novel surface Lewis acidic sites and/or Lewis basic sites. The ‘fixed’ surface lattice atoms near the constructed surface defects in a close proximity may be unbonded, which can avoid the formation of classic Lewis acid–base adjuncts due to the rigid crystal lattice. Such a configuration may activate the small inert molecules such as H 2 and CO 2 . Our hypothesis here is that the activation of inert molecules can be realized by rationally designed surface engineering and regulation on the structural defects of metal oxides to create novel FLP active sites. This possibility is illustrated by taking CeO 2 as an example in view of both the geometrical and electronic configurations ( Fig. 1 ). 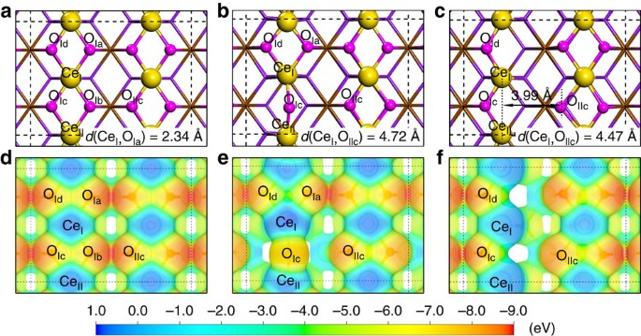Figure 1: Schematic images of concept for design of solid frustrated Lewis pairs in CeO2crystal structure. (a) Optimized structure of ideal CeO2(110). (b) Optimized structure of CeO2(110) with one oxygen vacancy. (c) Optimized structure of CeO2(110) with two adjacent oxygen vacancies. (d) Electron-density isosurface of ideal CeO2(110). (e) Electron-density isosurface of CeO2(110) with one oxygen vacancy. (f) Electron-density isosurface of CeO2(110) with two oxygen vacancies. The electron-density isosurfaces are plotted at 0.01ebohr−3. The colour bar represents the electrostatic potential scale. Figure 1: Schematic images of concept for design of solid frustrated Lewis pairs in CeO 2 crystal structure. ( a ) Optimized structure of ideal CeO 2 (110). ( b ) Optimized structure of CeO 2 (110) with one oxygen vacancy. ( c ) Optimized structure of CeO 2 (110) with two adjacent oxygen vacancies. ( d ) Electron-density isosurface of ideal CeO 2 (110). ( e ) Electron-density isosurface of CeO 2 (110) with one oxygen vacancy. ( f ) Electron-density isosurface of CeO 2 (110) with two oxygen vacancies. The electron-density isosurfaces are plotted at 0.01 e bohr −3 . The colour bar represents the electrostatic potential scale. Full size image Starting from the ideal CeO 2 (110) facet, the surface Ce and O form Lewis acid–base adjuncts ( Fig. 1a ). Two kinds of surface configurations, Ce I -O I(a ∼ d) and Ce I -O IIc , are identified on the ideal CeO 2 (110) surface. Ce I and O I(a ∼ d) are adjacent and contiguous to each other, forming a classic Lewis acid–base adjunct, whereas the unbonded Ce I and O IIc show a distance of 4.60 Å, which may deliver FLP-like activity. However, the electronic interactions between Ce I and its neighbouring O Ib will block the function of Ce I -O IIc pairs as shown in Fig. 1d . Therefore, the removal of oxygen atom directly linked with Ce I is the prerequisite to construct a pair of unbonded Lewis acid and base sites. When the O Ib atom is removed, two surface Ce atoms (including Ce I ) are reduced and one oxygen vacancy is produced, as demonstrated by the Bader charge population analysis of surface Ce ( Supplementary Table 1 ). After structural relaxation, the O Ic near the oxygen vacancy immigrates to the middle of the Ce I and Ce II , leading to Ce I being surrounded by three adjacent oxygen atoms ( Fig. 1b ). In this case, three types of configurations can be found including Ce I -O Ia/Id , Ce I -O Ic and Ce I -O IIc , of which the Ce I -O Ia/Id and Ce I -O Ic form classic Lewis acid–base adjuncts. The Ce I -O IIc with a distance of 4.72 Å falls in the domain of solid FLPs to activate small molecules but is still hindered by O Ic/Ia due to the electronic interaction between Ce I and O Ic/Ia ( Fig. 1e ). When the second surface oxygen (O Ia ) is removed, two oxygen vacancies and four reduced Ce cations (including Ce I and Ce II ) are generated ( Fig. 1c and Supplementary Table 1 ). The left oxygen O Ic and O Id will not migrate to the middle of two Ce cations. Thus, the reduced Ce cations (Ce I and Ce II ) and surface lattice oxygen (O IIc ) are independent Lewis acid and base, indicating that Ce I -O IIc and Ce II -O IIc may act as the solid FLPs ( Fig. 1c,f ), similar to molecular FLPs. In addition, a special FLP-like active site of two adjacent reduced surface Ce sites (Ce I and Ce II ) and lattice O IIc is constructed and denoted as (Ce I ,Ce II )-O IIc hereafter. Compared with Ce I -O IIc and Ce II -O IIc configurations, (Ce I ,Ce II )-O IIc with a shorter distance (3.99 Å) and stronger charge contraction by two adjacent reduced surface Ce cations is likely to deliver a higher capability to activate small molecules. On the other hand, the larger concentration of oxygen vacancy also increases the electron density of oxygen atoms (Bader charge analysis, Supplementary Table 1 ), suggesting the higher ability of oxygen to donate electrons. Bearing the above discussion in mind, it is possible to realize all-solid FLP catalysts of CeO 2 by regulating the surface defects. Similar to the CeO 2 (110) surface, the solid FLPs can also be constructed by removing surface oxygen atoms of the CeO 2 (100) surface. The surface oxygen atoms locate in the first atomic layer and surface cerium atoms sit in the second atomic layer on the ideal CeO 2 (100) surface ( Supplementary Figs 1a and 14b ). The Ce I -O Ia pair forms a classic Lewis acid–base adjunct with a distance of only 2.19 Å. Although the Ce I -O Ic pair has a distance of 4.41 Å, it fails to be a FLP as the blocking of O Ib next to Ce I ( Supplementary Fig. 1c ). Removal of O Ib can construct a FLP site, (Ce I ,Ce II )-O Ic with a distance of 3.95 Å ( Supplementary Fig. 1b,d ), similar to the solid FLP catalyst on the reduced CeO 2 (110) surface. However, the construction of surface FLP site cannot be realized by removing surface oxygen atoms on the CeO 2 (111) facet. Similar to the ideal CeO 2 (110) surface, two types of Lewis acid-base pairs, that is, Ce I -O Ic and Ce II -O IIc , are classic Lewis acid-base pairs on the ideal CeO 2 (111) surface. If one O atom (O Ic in Supplementary Fig. 2a ) is removed ( Supplementary Fig. 2b ), the O IIc atom is still surrounded by Ce II and Ce III without the formation of FLP ( Supplementary Fig. 2e ). Similarly, when two O atoms (O Ib and O Id in Supplementary Fig. 2a ) are removed ( Supplementary Fig. 2c ), O Ia and Ce I also cannot form FLPs owing to the blocking by Ce II * and Ce III * ( Supplementary Fig. 2f ). Therefore, the CeO 2 nanostructures with the mainly exposed (110) and (100) facets may possess high catalytic hydrogenation activity rising from the formation of the solid FLPs. Catalytic hydrogenation activity of PN- CeO 2 To explore the possibility of metal oxides as all-solid FLP catalysts, PN -CeO 2 with mainly exposed (110) and (100) facets, is selected as the model catalysts and hydrogenation of styrene is selected as a feature reaction. PN -CeO 2 has been previously reported with a high surface Ce 3+ fraction (30.8%) and a large concentration of oxygen vacancy [53] , [54] , [55] , [56] . Besides, the surface properties of PN -CeO 2 can be effectively regulated by post-treatment with well preserved structural features, providing a platform to investigate the correlation between the hydrogenation activity of ceria and their surface properties. PN -CeO 2 was synthesized through a two-step hydrothermal synthetic approach, in which nonporous nanorods ( Supplementary Fig. 3 ) with the mixed phases of Ce(OH) 3 and CeO 2 was obtained in the first-step hydrothermal process at 100 °C and porous nanorods with cubic fluorite structure were synthesized by dehydration/oxidation of precursor nanorods at the second hydrothermal treatment at 160 °C. Both bright-field and dark-field transmission electron microscopic (TEM) studies reveal a porous rod-like morphology with a dimension of ∼ 8 × 60 nm ( Fig. 2a,b ). X-ray diffraction (XRD) analysis confirms the precursor nanorods undergo the dehydration of the Ce(OH) 3 content being transformed into CeO 2 at 160 °C ( Supplementary Figs 3b and 4 ). High-resolution TEM (inset Fig. 2a ) image of PN -CeO 2 exhibits two kinds of lattice fringes of (220) and (200), which have respective inter-planar spacings of 0.191 and 0.275 nm. Similar to previous reports, the nanorods preferentially grow along [110] direction and are enclosed by (220) and (200) planes [57] . Derived from dark-field TEM images, the average pore size is 2.94±0.78 nm, which is similar as the average value of 2.2 nm obtained from the gas adsorption isotherms ( Supplementary Fig. 5a,c,d ). Surface area of PN -CeO 2 determined by Brunauer–Emmett–Teller analysis is 122 m 2 g −1 ( Supplementary Fig. 5b ). 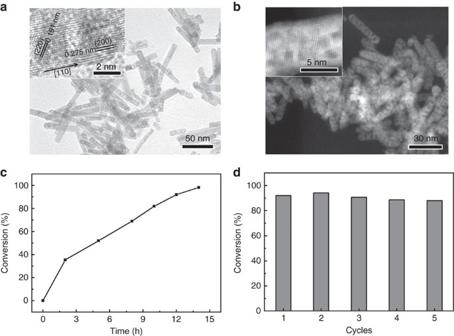Figure 2: Structural characterization and catalytic performance ofPN-CeO2catalysts for hydrogenation of styrene. (a) Bright-field TEM image ofPN-CeO2. Inset is the high resolution TEM image ofPN-CeO2. (b) Dark-field TEM image ofPN-CeO2. High resolution TEM image of inset displays a pore size of 2.94±0.78 nm. (c) Time course of styrene conversion catalysed byPN-CeO2. (d) Recyclability ofPN-CeO2catalysts for hydrogenation of styrene. Reaction conditions: styrene (1.0 mmol), toluene (0.5 ml) andPN-CeO2(20.0 mg) at 100 °C and 1.0 MPa H2pressure. Figure 2: Structural characterization and catalytic performance of PN -CeO 2 catalysts for hydrogenation of styrene. ( a ) Bright-field TEM image of PN -CeO 2 . Inset is the high resolution TEM image of PN -CeO 2 . ( b ) Dark-field TEM image of PN -CeO 2 . High resolution TEM image of inset displays a pore size of 2.94±0.78 nm. ( c ) Time course of styrene conversion catalysed by PN -CeO 2 . ( d ) Recyclability of PN -CeO 2 catalysts for hydrogenation of styrene. Reaction conditions: styrene (1.0 mmol), toluene (0.5 ml) and PN -CeO 2 (20.0 mg) at 100 °C and 1.0 MPa H 2 pressure. Full size image Initially, optimization of the reaction conditions for hydrogenation reaction catalysed by PN- CeO 2 is shown in Supplementary Table 2 . Despite the catalytic activity of PN- CeO 2 had been observed at a low temperature of 60 °C and low H 2 pressure of 0.2 MPa, an unsatisfied styrene conversion of 34.9% was delivered after 24 h reaction. Raising reaction temperature (100 °C) and H 2 pressure (1.0 MPa) realized the complete hydrogenation of styrene in 14 h successfully. Figure 2c shows time course of hydrogenation of styrene catalysed by PN- CeO 2 . The reaction proceeded continuously to reach 98.2% conversion of styrene in 14 h and afford >99.9% chemoselectivity towards ethylbenzene. After catalytic hydrogenation reaction, PN- CeO 2 were recovered by centrifugation and washed with ethanol for three times. Before reuse, the spent PN- CeO 2 catalysts were treated at 220 °C for 4 h under the argon protection. Afterwards, PN- CeO 2 can achieve five-time recyclability without any obvious catalytic degradation ( Fig. 2d ). The unaltered morphology, unchanged phase and almost no changed surface Ce 3+ fraction of the spent PN -CeO 2 illustrate their structural and catalytic stability during hydrogenation reactions ( Supplementary Fig. 6 ). Catalytic screening of various metal oxides Derived from the previous studies on the semi-hydrogenation of alkynes by ceria [47] , PN- CeO 2 with a high concentration of surface defects should inactive or even inert for hydrogenation of styrene. To understand the high catalytic activity of PN- CeO 2 in the current work, the catalytic activity of various metal oxides including acidic oxides, basic oxides and transition metal oxides for hydrogenation of styrene were also investigated under 100 °C and 1.0 MPa for 14 h. As presented in Fig. 3a , the typical acidic oxides (SiO 2 , Al 2 O 3 and SnO 2 ) delivered a very poor catalytic activity with styrene conversions below 1.4%. Poor catalytic activity of basic oxides (CaO, MgO and ZnO) was also observed. Meanwhile, the styrene conversions obtained from other common transition metal oxides, CuO, Fe 2 O 3 , NiO, MoO 3 and Co 3 O 4 , were below 0.8%, indicating their inertness for the hydrogenation of alkenes under the operated conditions. 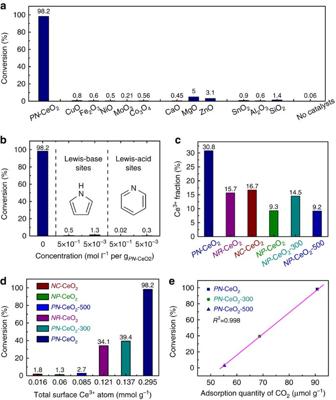Figure 3: Mechanism investigations on hydrogenation activity ofPN-CeO2. (a) Catalytic activity of various metal oxides for hydrogenation of styrene. (b) Influences of molecular Lewis-base or Lewis-acid on the catalytic activity ofPN-CeO2for hydrogenation of styrene. (c) Catalytic activity of nanoceria for hydrogenation of styrene. (d) Effects of the total surface Ce3+atom number for hydrogenation of styrene. (e) Correlation between conversion of styrene and adsorption quantity of CO2on CeO2catalyst. Reaction conditions: styrene (1.0 mmol), toluene (0.5 ml) and catalysts (20.0 mg) at 100 °C and 1.0 MPa H2pressure for 14 h. Figure 3: Mechanism investigations on hydrogenation activity of PN -CeO 2 . ( a ) Catalytic activity of various metal oxides for hydrogenation of styrene. ( b ) Influences of molecular Lewis-base or Lewis-acid on the catalytic activity of PN -CeO 2 for hydrogenation of styrene. ( c ) Catalytic activity of nanoceria for hydrogenation of styrene. ( d ) Effects of the total surface Ce 3+ atom number for hydrogenation of styrene. ( e ) Correlation between conversion of styrene and adsorption quantity of CO 2 on CeO 2 catalyst. Reaction conditions: styrene (1.0 mmol), toluene (0.5 ml) and catalysts (20.0 mg) at 100 °C and 1.0 MPa H 2 pressure for 14 h. Full size image Control experiments ( Fig. 3a ) indicated that the hydrogenation reaction of styrene could not happen in the absence of PN -CeO 2 , indicating the nature catalytic ability of PN -CeO 2 . The major difference between PN -CeO 2 and other metal oxides is the coexistence of Lewis acidic and basic sites in high concentrations for PN -CeO 2 . Therefore, the survey of metal oxides for hydrogenation of styrene indicates that the absence of either acidic or basic sites on the surface of metal oxides results in near complete deactivation for the hydrogenation of alkenes. To further confirm the necessity of the co-existence of Lewis acidic and basic sites of PN -CeO 2 in current catalytic system, hydrogenation of styrene was performed in the presence of other molecular Lewis acid or base during the catalytic process. The Lewis base pyridine and Lewis acid pyrrole as common molecules are generally used to confirm the presence of Lewis acidic and basic sites for metal oxides, respectively. As a strong base pyridine (strong acid pyrrole) can be able to absorb on the Lewis acidic (Lewis basic) sites of PN -CeO 2 immediately, when they are added to the reaction solution. Therefore, the FLPs can be effectively blocked by the pyridine and pyrrole molecule. As shown in Fig. 3b , addition of trace amount of either Lewis base pyridine or Lewis acid pyrrole completely terminated the hydrogenation reactions due to the blockage of surface Lewis acidic or basic sites by those small molecules, respectively, similar to that of molecular FLPs [58] , [59] . Trace amount of pyridine/pyrrole molecules were adsorbed on the surface Lewis acidic/basic sites of CeO 2 , leading to a low possibility for the formation of surface FLP sites in the aspect of population of adjacent surface Ce 3+ . The blockage of either Lewis basic sites or Lewis acidic sites of PN -CeO 2 leads to the deactivated hydrogenation of alkenes, revealing that the coexistence of Lewis acidic and basic sites on the surface of PN -CeO 2 are essential to activate H–H bond and achieve high activity in the current system. Role of surface defects of PN -CeO 2 for hydrogenation For the semi-hydrogenation of alkynes by ceria, hydrogen dissociative adsorption on surface oxygen leads to the formation of two surface –OH groups and dissociation of C–H bond of R−C≡C−H on the adjacent surface Ce and O atoms [49] . In those studies, three points were outlined: (1) the obtained alkenes cannot be further reduced into alkanes; (2) experimental results suggest that the hydrogen activation process is the rate-limiting step due to the poor ability of ceria to cleave H−H bond; (3) the catalytic activity of ceria can be significantly decreased in the presence of large amount of surface defects. Followed by the literature reports, PN -CeO 2 with a high surface concentration of oxygen vacancy should deliver a poor catalytic activity for hydrogenation reactions. In fact, PN -CeO 2 indeed shows a very high catalytic activity for styrene hydrogenation, suggesting a different catalytic mechanism for the current work. Besides, both alkenes and alkynes can be reduced by PN -CeO 2 under much mild conditions (see Discussion below), also revealing an alternative catalytic pathway for hydrogen activation and subsequent hydrogenation. To explore the roles of surface defects of ceria, hydrogenation of styrene was also performed for ceria nanoparticles ( NP -CeO 2 ) with a surface Ce 3+ fraction of 9.3% ( Supplementary Fig. 7 ), ceria nanocubes ( NC -CeO 2 ) with a surface Ce 3+ fraction of 16.7% ( Supplementary Fig. 8 ) and non-porous ceria nanorods ( NR -CeO 2 ) with a surface Ce 3+ fraction of 15.7% ( Supplementary Fig. 9 ). The conversions of styrene were only 1.3%, 1.8% and 34.1% for NP -CeO 2 , NC -CeO 2 and NR -CeO 2 under the identical reaction conditions of those catalysed by PN -CeO 2 for 14 h, respectively ( Fig. 3d ). The surface area of 98 m 2 g −1 for NR -CeO 2 is close to that of PN -CeO 2 of 122 m 2 g −1 ( Supplementary Table 3 ), indicating surface area is not the critical factor to determine their difference in their catalytic activity for hydrogenation of alkenes. The high consistence between the surface Ce 3+ fractions and the catalytic activity of ceria reveals that the hydrogenation activity of ceria is determined by the abundance of the surface defect sites. As predicted from the theoretical calculations, it is also possible to create the surface FLP sites on CeO 2 (100) surface. However, the catalytic activity of NC -CeO 2 was much lower than that of PN -CeO 2 . Considering the small surface area of NC -CeO 2 , we also performed the hydrogenation of styrene by 200 mg NC -CeO 2 with the comparable surface area to that of 20 mg PN -CeO 2 under the identical conditions. A very low styrene conversion of 5.3% was observed, which could be attributed to the low concentration of surface defects of NC -CeO 2 with a Ce 3+ fraction of 16.7%. The results further confirm that the concentration of surface defects is the main factor to construct large amount of surface FLP sites without regard to the morphology of CeO 2 catalysts. Hydrogenation performance of NR -CeO 2 (20 mg) and NC -CeO 2 (200 mg) catalysts suggested that the catalytic activity of FLP sites on CeO 2 (110) was higher than that of CeO 2 (100) with similar surface Ce 3+ fractions ( Fig. 3c,d ). It can be attributed to the different steric configuration of FLP sites on CeO 2 (110) and CeO 2 (100). Both the acidic and basic sites of the constructed FLP sites on CeO 2 (110) are in the top atomic layer ( Fig. 1c,f and Supplementary Fig. 14a ), whereas the basic sites (O atoms) on CeO 2 (100) are in the top atomic layer with the second atomic layer of the acidic sites (Ce atoms) ( Supplementary Figs 1d and 14b ). Both two configurations can effectively activate hydrogen molecule. However, styrene can encounter less steric hindrance when reacting with the intermediate of heterolysis of H 2 at the FLP sites on CeO 2 (110). Besides, due to the high surface energy, oxygen atoms of CeO 2 (100) is more prone to diffuse on surface than that of CeO 2 (110) [60] . This diffuse of oxygen atoms (basic sites) can break the steric encumbered structures of FLP sites, leading to the decrease in activity of FLP sites or even the formation of classic acid-base adduct. Thus, the FLP sites on CeO 2 (100) are less stable than those on CeO 2 (110), indicating that the stability of FLP sites could be another factor in the decrease of activity on CeO 2 (100) surface. The surface Ce 3+ fractions of PN -CeO 2 were effectively reduced from 30.8% of as-synthesized catalysts to 14.5 and 9.2% ( Fig. 3c and Supplementary Fig. 10 ), when PN -CeO 2 was treated at 300 °C (obtained PN -CeO 2 -300 catalysts) and 500 °C (obtained PN -CeO 2 -500 catalysts) in air for 8 h, respectively. The calcinated PN -CeO 2 preserved the porous morphology ( Supplementary Fig. 11 ), as well as their surface areas ( Supplementary Table 3 ). After calcination, the obtained PN -CeO 2 catalysts were immediately used for hydrogenation of styrene under the same conditions. The 39.4% and 2.7% conversions of styrene were yielded with PN -CeO 2 -300 and PN -CeO 2 -500, respectively. The decreased catalytic activity can only be attributed to their decreased concentration of surface oxygen vacancy due to the high temperature annealing at 300 and 500 °C in air. On the other hand, the PN -CeO 2 was reduced under 10% H 2 /Ar at 200 °C for 2 h and then transferred from the reducing atmosphere to the hydrogenation system immediately. The exposure of the reduced PN -CeO 2 to air was controlled 5 min to minimize the re-oxidation of the reduced catalysts. The catalytic activity for reduced PN -CeO 2 also enhanced from 69.1% to 86.4% after 8 h reaction ( Supplementary Fig. 12 ). The enhanced catalytic activity can be attributed to the increased concentration of surface oxygen vacancy, leading to an increased possibility to construct more surface FLP sites. Therefore, the parallel experiments further strengthen the evidence linking the concentration of surface oxygen vacancy of PN -CeO 2 with their catalytic activity for hydrogenation of alkenes. The decreased hydrogenation activity of PN -CeO 2 -300 and PN -CeO 2 -500 can be further revealed from the temperature-programmed hydrogen desorption (H 2 -TPD) tests. All PN -CeO 2 catalysts were exposed to H 2 at 50 °C and the weakly physisorbed hydrogen was removed by flushing Ar for 20 min. A desorption peak at 190 °C was observed for all PN -CeO 2 catalysts ( Supplementary Fig. 13 ), indicating a strong interaction between H 2 and PN -CeO 2 . With the increase of calcination temperature, the decreased peak intensities demonstrated the reduced amount of activated hydrogen on PN -CeO 2 -300 and PN -CeO 2 -500. Therefore, the decreased catalytic activity of the calcined PN -CeO 2 was delivered for styrene hydrogenation. Mechanism investigations All control experiments strongly suggest that the coexistence of Lewis acidic and basic sites plays extremely important roles in activating hydrogen at mild conditions and realising their high catalytic activity for hydrogenation reactions. The results are totally different to the catalytic mechanism of the semi-hydrogenation of alkynes by ceria [47] , [48] , [49] . In Fig. 1 , we have illustrated that it is possible to create FLP active sites through regulations on the surface defects of CeO 2 (110). In general, the key features of organic molecules FLP catalysts are defined as the independent Lewis acid and base in the presence of sterically substituents on Lewis acid and base to preclude the formation of the classical Lewis acid–base adducts [30] , [61] . Addition of any other small Lewis acid or base molecules results in the formation of adducts and completely blocks the catalytic activity of FLP catalysts during the catalytic process [9] , [12] , [28] . On the basis of the known essentiality of molecular FLP catalysts and a strong correlation between the hydrogenation activity and surface properties of PN -CeO 2 with coexistence of Lewis acid and base in current system, it’s logical to rationalize the PN -CeO 2 as all-solid FLP catalysts. The analogous aspects of molecular FLP catalysts and PN -CeO 2 are listed: (1) independent surface Lewis acidic and basic sites of PN -CeO 2 ( Fig. 1c ); (2) close proximity (4 ∼ 5 Å) between surface Lewis acidic site and basic site for activation or splitting of small molecules; and (3) completely quenched hydrogenation activity with addition of other Lewis acids or bases. To support the aforementioned conclusions, DFT calculations using the Vienna Ab-initio Simulation Package [62] , [63] , [64] were performed to investigate the adsorption and activation of hydrogen on the CeO 2 (110) surface. For ideal CeO 2 (110) ( Supplementary Fig. 14a ), hydrogen molecule prefers to be adsorbed at the top site of Ce I ( Fig. 4a ) or classic acid–base site ( Fig. 4b ) with weak adsorption energies of −0.06 eV, in consistence with previous studies [65] , [66] . The H–H bond length of the weakly adsorbed H 2 is 0.75 and 0.76 Å for the two adsorption configurations, respectively. These values are close to that of gas phase H 2 (0.75 Å), suggesting that H 2 is difficult to be activated on ideal CeO 2 (110). The Bader charge populations of the physisorbed H 2 ( Fig. 4a,b ) further indicate that H 2 is slightly polarized and hardly activated on ideal CeO 2 (110). With one oxygen vacancy constructed on CeO 2 (110), the adsorption and activation of H 2 is still poor on both Ce I -O Ic ( Fig. 4c , −0.06 eV) and Ce I -O IIc sites ( Fig. 4d , −0.04 eV), which is further evidenced by the long distance ( ∼ 3.0 Å) between H 2 and CeO 2 (110) surface and the similar H−H bond length of adsorbed H 2 to that of gas-phase H 2 . For the surface with two adjacent oxygen vacancies, H 2 preferentially adsorbs at the created solid FLP site (Ce I ,Ce II )-O IIc ( Fig. 4f ) rather than on the top site of the unsaturated Ce atom ( Fig. 4e ). The results reveal the easy activation of H 2 molecule at the site of (Ce I ,Ce II )-O IIc : (1) a relatively larger adsorption energy of H 2 of −0.13 eV ( Fig. 4f ). (2) A significantly elongated H−H bond length of 0.80 Å. (3) A shorter distance between H 2 and the CeO 2 (110) than those in other adsorption configurations ( Fig. 4a-e ). The distance between one hydrogen atom of H 2 and the base site of solid FLPs is only 1.89 Å. (4) A larger polarization of H−H bond due to the electrostatic interactions between the FLPs and H 2 , as indicated in the Bader charge of −0.16 e and +0.11 e for two hydrogen atoms ( Fig. 4f ). The aforementioned aspects strongly suggest that the novel solid FLP site constructed by two Ce cations and one O anion is more effective in H 2 adsorption and activation than the classic acid–base adjuncts. 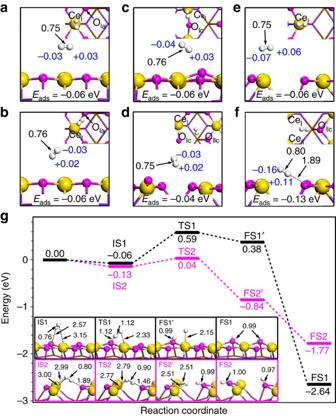Figure 4: The H2adsorption and dissociation pathways on the surface ofPN-CeO2. The optimized structures of H2adsorption on (a) CeIatom of ideal CeO2(110); (b) CeI-OIapair of ideal CeO2(110); (c) CeI-OIcpair of CeO2(110) with one oxygen vacancy; (d) CeI-OIIcpair of CeO2(110) with one oxygen vacancy; (e) CeIatom of CeO2(110) with two oxygen vacancies; and (f) (CeI,CeII)-OIIcpair of CeO2(110) with two oxygen vacancies in both top (inset) and side views. The adsorption energies (Eads), the bond distances (in Å) colored in black, and the Bader charge population (ine) colored in blue are also shown. (g) Energy profiles for H2dissociation on ideal CeO2(110) in black curve and CeO2(110) with two oxygen vacancies in red curves. The optimized structures of initial states (IS), transition states (TS) and final states (FS) are labeled with bond distance (in Å). The zero energy reference corresponds for the sum energy of H2in the gas phase and the corresponding clean CeO2surfaces. Figure 4: The H 2 adsorption and dissociation pathways on the surface of PN -CeO 2 . The optimized structures of H 2 adsorption on ( a ) Ce I atom of ideal CeO 2 (110); ( b ) Ce I -O Ia pair of ideal CeO 2 (110); ( c ) Ce I -O Ic pair of CeO 2 (110) with one oxygen vacancy; ( d ) Ce I -O IIc pair of CeO 2 (110) with one oxygen vacancy; ( e ) Ce I atom of CeO 2 (110) with two oxygen vacancies; and ( f ) (Ce I ,Ce II )-O IIc pair of CeO 2 (110) with two oxygen vacancies in both top (inset) and side views. The adsorption energies ( E ads ), the bond distances (in Å) colored in black, and the Bader charge population (in e ) colored in blue are also shown. ( g ) Energy profiles for H 2 dissociation on ideal CeO 2 (110) in black curve and CeO 2 (110) with two oxygen vacancies in red curves. The optimized structures of initial states (IS), transition states (TS) and final states (FS) are labeled with bond distance (in Å). The zero energy reference corresponds for the sum energy of H 2 in the gas phase and the corresponding clean CeO 2 surfaces. Full size image To further confirm the high activity of such a constructed solid FLP site towards the activation of small molecules, the dissociative activation of H 2 is investigated on the ideal CeO 2 (110) and reduced CeO 2 (110) surface in the presence of (Ce I ,Ce II )-O IIc . From the energy profile depicted by Fig. 4g (black curve), the dissociation of H 2 on ideal CeO 2 (110) starts from a physisorbed state (IS1) and surpasses an activation barrier of 0.65 eV to reach a dissociated state (FS1’). In FS1’, the dissociated hydrogen bound to Ce site is meta-stable and readily diffuses to nearby surface oxygen, leading to the formation of a more stable FS1. The H 2 dissociation on CeO 2 (110) with the solid FLP active sites experiences a similar process, which also starts from a physisorbed state. Noticeably, the dissociation barrier is only 0.17 eV on the constructed FLP site, which is 0.48 eV lower than that on ideal CeO 2 (110). Moreover, the dissociation of H 2 on solid FLPs (from IS2 to FS2’) is exothermic by 0.71 eV in contrast to the endothermic energy (0.44 eV, from IS1 to FS1’) on ideal CeO 2 (110). Both kinetic and thermodynamic results suggest that the dissociative activation of H 2 is more favourable on the reduced CeO 2 (110) with active FLP sites. The dissociated hydrogen anchored at the Ce site (FS2’) can immigrate to an adjacent oxygen to form FS2 with an exothermic energy of 0.93 eV. It is worth noting that FS2 is less stable than FS1, despite two hydrogen atoms are both adsorbed at surface oxygen in two configurations. The calculations suggest that the O–H bond in FS2 is weaker than that in FS1. The weakness of O–H bond is attributed to the enhanced basicity of oxygen on the reduced CeO 2 (110), which is detrimental to the adsorption of H according to the rules of Lewis acid-base pairs on oxide surfaces [67] . Fortunately, the less stable O–H bonds are expected to benefit the subsequent hydrogenation reactions. Derived from DFT calculations, CeO 2 nanorods with a high concentration of surface oxygen defects deliver a high possibility to create surface (Ce I ,Ce II )-O IIc FLP sites, yield an enhanced capability of dissociation of H 2 and improve their catalytic activity for hydrogenation of styrene. The calculation results ( Fig. 4 ) are highly consistent with experiments ( Fig. 3 ), supporting the solid FLP-like activity of PN -CeO 2 regulated and constructed by the surface oxygen defects as illustrated in Fig. 1 . To further confirm this conclusion, the correlation between catalytic activity and the concentration of the surface oxygen vacancy of CeO 2 were studied through the TPD of CO 2 on the various PN -CeO 2 - T catalysts. The annealed PN -CeO 2 at 300 and 500 °C exhibited the identical morphological features to those of as-synthesized PN -CeO 2 ( Supplementary Fig. 11 ). Importantly, the PN -CeO 2 -300 (120 m 2 g −1 ) and PN -CeO 2 -500 (117 m 2 g −1 ) showed similar surface areas to that of as-synthesized PN -CeO 2 (122 m 2 g −1 ). Thus, such a system provides a straightforward way to understand the correlations between the acidity/basicity of PN -CeO 2 and their catalytic activity. In previous reports, CO 2 as a Lewis acid can bind with O 2− surface ions forming carbonate species with various anchoring structures (bridged, bidentate, monodentate and polydentate) [50] . Furthermore, the presence of oxygen vacancy on CeO 2 surface can make a strong interaction with CO 2 and thus enhance its surface basicity [58] . The surface adsorption quantity of CO 2 is the highest on PN -CeO 2 (90.7 μmol g −1 ), followed by PN -CeO 2 -300 (68.7 μmol g −1 ), and the least on PN -CeO 2 -500 (55.2 μmol g −1 ) from the CO 2 -TPD results ( Supplementary Fig. 15 and Supplementary Table 4 ). The reduced surface basic sites mainly derived from the obviously decreased medium and strong basic sites, which indicated the decreased amount of surface oxygen vacancy. Meanwhile, the conversions of styrene showed a near linear decrease with the decreased adsorption quantity of CO 2 on various PN -CeO 2 catalysts ( Fig. 3e , R 2 =0.998). Results further demonstrate the importance of the surface abundance of defects in CeO 2 catalysts to construct the surface FLP sites once more. The correlation between the concentration of oxygen vacancy and their catalytic activity is further investigated with Raman spectra analysis. The concentration of oxygen vacancy is indexed by the ratio of the integrated peak area under the bands at 460 cm −1 (vibrational mode of CeO 2 fluorite structure) and 600 cm −1 (oxygen vacancy) of the Raman spectra of PN -CeO 2 annealed at various temperatures ( Supplementary Fig. 16 ) [28] . The decrease in the A 600 /A 460 with the increased calcination temperature indicates a decrease in the number of oxygen vacancy, as well as the surface Ce 3+ fraction. Thus, high temperature treatment on PN -CeO 2 leads to the decrease in the number of FLPs sites. Therefore, it is not surprising to observe an obviously decreased conversion of styrene with PN -CeO 2 -300 and PN -CeO 2 -500; even they have almost the same surface areas ( Supplementary Table 3 ). The conversion of styrene as a function of total surface Ce 3+ species ( Fig. 3d ) and the concentration of oxygen vacancy ( Fig. 3e and Supplementary Fig. 16b ) indicate that the abundance of surface defects is important for the construction of FLP active sites on PN -CeO 2 . The high concentration of surface defects introduces a high possibility to form the surface FLP sites as shown in Fig. 1c . Both theoretical calculations and experimental results illustrate that the FLP active sites in PN -CeO 2 are created by regulations on their surface properties. Hydrogenation scope of alkenes The scope of hydrogenation reactions catalysed by PN -CeO 2 was demonstrated in Table 1 . When the electron-donating groups of methyl (–CH 3 ), tertiary butyl (–C(CH 3 ) 3 ) and methoxy (–OCH 3 ) were introduced in styrene, the reactant conversions of 99.1, 98.1 and 99% were yielded under 0.6, 0.6 and 1.0 MPa H 2 pressure, respectively (Entry 1, 2 and 3). However, the catalytic hydrogenation activity of PN -CeO 2 was obviously decreased in the presence of electron-drawing groups in the substrates. The introduction of –Br and –Cl afforded the conversions of 98.5% and 79.5% under 1.0 MPa H 2 pressure for 20 h, respectively (Entry 4 and 5). It can be attributed to the decreased electronic density of vinyl group in the presence of electron-drawing groups in benzene ring. The hydrogenation of cyclooctene into cyclooctane reached a conversion of 90.5% under 1.0 MPa H 2 pressure for 20 h (Entry 6). When the H at α or β site of vinyl is replace by other groups, the catalytic activity of PN -CeO 2 for hydrogenation of vinyl is also decreased due to steric hindrance. Compared to 56.3% conversion of α-methylstyrene under 1.0 MPa H 2 for 20 h (Entry 7), trans -stibene and cis -stilbene only reached 10.3% and 8.9% conversions under the same reaction conditions, respectively (Entry 8 and 9). Table 1 Scope of PN -CeO 2 for catalytic hydrogenation of alkenes * . Full size table In light of both experimental and theoretical investigations, the introduction of oxygen vacancy is very important in the formation of FLP active sites for PN -CeO 2 . When alkenes include oxygen-containing groups, the blockage of the surface FLP active sites on PN -CeO 2 may happen due to the strong adsorption of oxygen at the surface defects. Thus, the catalytic activity of PN -CeO 2 for those molecules can be reduced or completely depressed. As shown in Table 1 (Entry 10 and 11), trans -cinnamaldehyde and allylacetone in the presence of formyl or ketone groups only yielded very low reactant conversions of 21.7% and 12.8%, respectively, despite a high chemoselectivity for olefine products (>99.9%). Owing to the strong interaction between –OH or –NO 2 groups and surface defects of PN -CeO 2 , the activity of FLPs was shielded with 4-hydroxystyrene and 4-nitrostyrene, affording very low conversions (<6%, Entry 12 and 13). There results further support the solid FLP catalytic behaviour of PN -CeO 2 for hydrogenation reactions. Hydrogenation scope of alkynes Ceria has shown the ability to selectively semi-hydrogenated alkynes into olefins [49] . Herein, hydrogenation of various alkynyl substrates was also evaluated with PN -CeO 2 ( Table 2 ). For hydrogenation of phenylacetylene, the conversion was increased from 55.8 to 100% with the increase of H 2 pressure from 1.0 to 3.0 MPa within 14 h (Entries 14 and 15). However, the selectivity towards styrene was decreased from 95.8 to 32.6% (Entries 14 and 15). By contrast, the selectivity of ethylbenzene was increased from 4.2 to 67.4% (Entry 14 and 15). Only ethylbenzene was obtained with the extended reaction time (Entry 16). The presence of electron-donating methyl group in phenylacetylene yielded 100% conversion under 3.0 MPa H 2 pressure but a poor chemoselectivity of 75.2% into 4-methylstyrene ( Table 2 , Entry 17). For 4-methoxy phenylacetylene, similar catalytic behaviour was observed with a 84.7% selectivity of olefin for the conversion of 100% under 3.0 MPa H 2 pressure at 100 °C (Entry 18). Introducing the electron-drawing substituents on phenylacetylene such as –Br and –Cl, the catalytic activity was reduced, as the low conversions of 50% and 13.7% were yielded for 4-bromo phenylacetylene and 4-chloro phenylacetylene under a H 2 pressure of 3.0 MPa and a temperature of 100 °C for 14 h, respectively (Entries 19 and 20). For 4-phenyl-1-butyne, 38.9% conversion and 100% selectivity towards olefin products were achieved under 3.0 MPa H 2 pressure for 14 h reaction (Entry 21). The catalytic activity of PN -CeO 2 was also decreased when the alkynes in the presence of the steric substituents. Under 3.0 MPa H 2 pressure, hydrogenation of diphenylacetylene only afforded a 13.8% conversion after 20 h reaction (Entry 22). The products of hydrogenation were a mixture of trans -stilbene and cis -stilbene with the chemoselectivity of 51.3% and 48.7%, respectively (Entry 23). Table 2 Scope of PN -CeO 2 for catalytic hydrogenation of alkynes * . Full size table In summary, we design all-solid metal oxide FLP catalysts through regulations on the surface properties of ceria. As demonstrated by both experimental and theoretical results, PN -CeO 2 with a high concentration of surface defects exhibits the FLP catalytic behaviour for the efficient hydrogenation of alkenes and alkynes with a wide scope. The high density of surface-bound defects is critical to generate the independent surface Lewis acidic and basic sites, construct the surface FLP pair of (Ce I ,Ce II )-O IIc ( Fig. 1c ) and improve their capability for H 2 activation with a low activation barrier of 0.17 eV. The capability to hydrogenate alkynes into alkanes further confirms the high hydrogenation activity of PN -CeO 2 . The current progress provides a new concept on the structurally correlated catalytic activity of ceria for hydrogenation reactions, which is important for the modern catalyst design. With the ease of preparation, such PN -CeO 2 as the active components in various hydrogenation reactions may be envisioned and so are their ultimate industrial applications. Preparation of PN -CeO 2 catalysts Aqueous solutions of Ce(NO 3 ) 3 ·6H 2 O (1.736 g in 10 ml of deionized water) [53] and NaOH (19.2 g in 70 ml of deionized water) were mixed slowly. With continuous stirring, the mixture was aged for 30 min before the reaction continued at 100 °C for 24 h in a temperature-controlled electric oven. The reaction mixture was then cooled naturally to room temperature. The products were collected by centrifugation, thoroughly washed with deionized water, and then air-dried at 60 °C. Hydrothermal treatment of this precursor product at 160 °C for 12 h afforded the formation of PN -CeO 2 . Characterizations The catalysts were characterized by powder XRD. The XRD patterns with diffraction intensity versus 2 θ were recorded in a Shimadzu X-ray diffractometer (Model 6000) using Cu K α radiation. TEM studies were conducted on the Hitachi HT-7700 with an accelerating voltage of 120 kV. High-resolution and dark-field TEM images were acquired from the Tecnai G2 F20 S-twin TEM at 200 kV. Surface area was measured by N 2 physisorption (Micromeritics, ASAP 2020 HD88) based on Brunauer–Emmet–Teller method. X-ray photoelectron spectroscopy were acquired using a Thermo Electron Model K-Alpha with Al K α as the excitation source. Catalytic hydrogenation reactions For a typical catalytic reaction, 1.0 mmol of substrate and 20.0 mg of catalysts were mixed in 0.5 ml of toluene. The reactions were performed in the autoclave charged with hydrogen with various pressures at the desired reaction temperature. The products were analysed by gas chromatography–mass spectrometry and gas chromatography with m-xylene as the internal standard. Data availability Data supporting the findings of this study are available within the article (and its Supplementary Information files) and from the corresponding author on reasonable request. How to cite this article: Zhang, S. et al . Solid frustrated-Lewis-pair catalysts constructed by regulations on surface defects of porous nanorods of CeO 2 . Nat. Commun. 8, 15266 doi: 10.1038/ncomms15266 (2017). Publisher’s note : Springer Nature remains neutral with regard to jurisdictional claims in published maps and institutional affiliations.